Deciphering the scaling of single-molecule interactions using Jarzynski’s equality Unravelling the complexity of the macroscopic world relies on understanding the scaling of single-molecule interactions towards integral macroscopic interactions. Here, we demonstrate the scaling of single acid–amine interactions through a synergistic experimental approach combining macroscopic surface forces apparatus experiments and single-molecule force spectroscopy. This experimental framework is ideal for testing the well-renowned Jarzynski’s equality, which relates work performed under non-equilibrium conditions with equilibrium free energy. Macroscopic equilibrium measurements scale linearly with the number density of interfacial bonds, providing acid–amine interaction energies of 10.9±0.2 kT. Irrespective of how far from equilibrium single-molecule experiments are performed, the Jarzynski’s free energy converges to 11±1 kT. Our results validate the applicability of Jarzynski’s equality to unravel the scaling of non-equilibrium single-molecule experiments to scenarios where large numbers of molecules interacts simultaneously in equilibrium. The developed scaling strategy predicts large-scale properties such as adhesion or cell–cell interactions on the basis of single-molecule measurements. Understanding how specific molecular interactions and molecular adhesion scale with increasing number densities of simultaneously interacting functionalities is vital to understanding the macroscopic outcome and design rules of molecular systems for a wide range of living and engineering structures. For example, in biological and biomedical systems, a large number of bonds interacting in parallel mediate cell-adhesion [1] cell-surface interactions [2] or bio-adhesion in marine environments [3] and tissue gluing [4] . Also in technological systems such as complex glues, a number of specific functionalities is combined to promote adhesion on the macroscopic scale without a detailed understanding for how adhesion evolves from the molecular level [5] , [6] . Deciphering macroscopic equilibrated interaction energies on the basis of experimentally measured single-molecular interactions is a largely unexplored field and demands systematic investigations to unravel the scaling of inherently non-equilibrium single-molecule dynamics to thermodynamically averaged interactions on a macroscopic scale. Single-molecule atomic force microscope experiments (SM-AFM) are now well established to measure unbinding/binding dynamics of protein unfolding [7] , [8] and specific and non-specific surface binding of single macromolecules [9] , [10] . Complementary surface forces apparatus (SFA) experiments have been extensively used to study equilibrated thermodynamic interaction forces at macroscopic contacts between surfaces providing specific interaction sites [11] , [12] , [13] , [14] . Here we show how using both techniques provides the ideal experimental framework for comparing non-equilibrium single-molecule force spectroscopy with macroscopic interaction energy measurements, which are thermodynamically averaged over a large number of simultaneously interacting single molecules. We show how a macroscopic equilibrated interaction energy results from the fluctuations of work measured for non-equilibrated single-molecular interactions, providing an experimental proof of Jarzynski’s equality [15] , [16] . 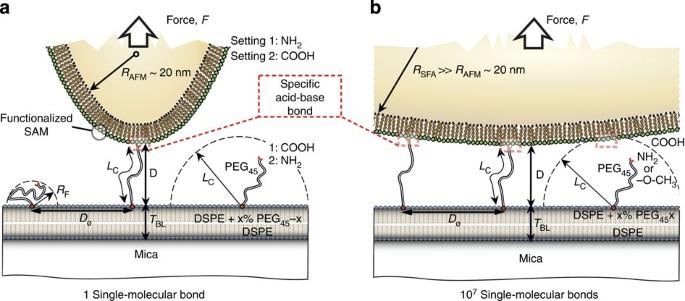Figure 1: Schematic of the experimental model systems. (a) In SM-AFM experiments a functionalized SAM (that is, in setting 1: NH2; or in setting 2: COOH) is used to ‘fish’ for complementary (that is, COOH or NH2) end-functionalities of end-grafted PEG-tethers extending from a lipid bilayer. (b) Complementary, macro-scale SFA measurements are used to probe the same molecularly designed systems with much larger contact area and hence a number of up to 107single-molecular bonds interacting simultaneously. Variation of the coverage Γ allows varying number densities of end-functionalized PEG45–X (with X=–NH2or –O–CH3) tethers and hence potentially formed molecular bonds, as well as adjustment of the average distancesDφbetween the tethered functional groups. Experimental approach Figure 1 shows a schematic of the designed experimental approach. Using SM-AFM and macroscopic SFA force versus distance measurements, we study the specific acid–base interaction between a carboxylic acid and an amine functionality. As exemplified in Fig. 1a , gold-coated SM-AFM tips modified with an end-functionalized self-assembled monolayer were probed against complementary end-functionalized and individualized polyethylene glycol (PEG) molecules extending from a lipid bilayer surfaces. For SFA, we studied the interaction energies of both amine-end functionalized and non-specifically functionalized lipid bilayers with varying concentrations facing a carboxylic acid end-functionalized SAM deposited on molecularly smooth gold surface ( Fig. 1b ). This complementary setup provides a means to individualize molecules for SM-AFM measurements with typical tip radii of R AFM ~20–30 nm. Likewise, one can study the scaling of macroscopic interaction energies based on exactly controlled number densities of formed acid–base bindings using SFA experiments with typical contact radii of R SFA ~1.5–2.5 cm. As such, our approach provides direct and complementary access to studying a given molecular bond from non-equilibrated single-molecule interactions up to equilibrium interactions of ~10 7 molecules interacting simultaneously over typical SFA contact areas of 100–1,000 μm 2 . Figure 1: Schematic of the experimental model systems. ( a ) In SM-AFM experiments a functionalized SAM (that is, in setting 1: NH 2 ; or in setting 2: COOH) is used to ‘fish’ for complementary (that is, COOH or NH 2 ) end-functionalities of end-grafted PEG-tethers extending from a lipid bilayer. ( b ) Complementary, macro-scale SFA measurements are used to probe the same molecularly designed systems with much larger contact area and hence a number of up to 10 7 single-molecular bonds interacting simultaneously. Variation of the coverage Γ allows varying number densities of end-functionalized PEG 45 –X (with X=–NH 2 or –O–CH 3 ) tethers and hence potentially formed molecular bonds, as well as adjustment of the average distances D φ between the tethered functional groups. 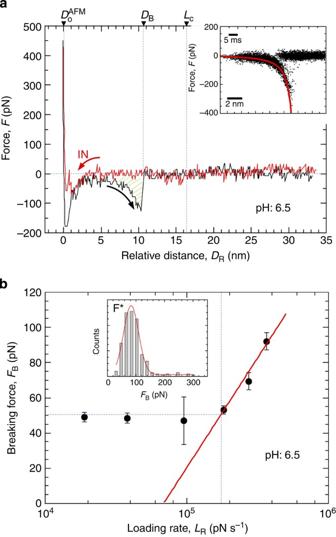Figure 2: Single-molecule force-induced rupture and force spectrum. (a) Typical non-equilibrium single-molecule rupture event measured in 1 mM NaCl, pH 6.5 at a pulling speedvp=0.25 μm s−1. The approach and retract curves are indicated. The AFM zero distance, the distance to bond breakingDBas well as the contour length,Lc(16.43 nm) of the used PEG tethers are indicated. Inset: About 100 pulling trajectories aligned with respect to pulling time using the best WLC-fit (red line, with persistence length as 3.65 Å). The scale bars are 2 nm and 5 ms. (b) Dynamic force spectra showing the logarithmic loading rate (LR=vpk) dependency of the unbinding force at pH=6.5. The near-equilibrium unbinding is visualized as a plateau for loading rates <105pN s−1. Non-equilibrium binding regimes are fit to the Bell–Evan’s equation as indicated by the solid line. The error bars represent s.e.m. Inset: histogram of breaking forces fitted to a Gaussian to extract the most probable unbinding force, F*. Full size image AFM single-molecule force spectroscopy Figure 2a shows a typical force–distance profile characterizing an unbinding event measured in SM-AFM. These events accounted to 20–60% of the total measured events in each set of measurement depending on specific configuration as well as pulling velocity, and are the key signatures of single-bond breaking under non-equilibrium conditions. Other observed events consisted of mostly non-specific adhesion as well as a small number of lipid pluck-out, bilayer poke-in and PEG desorption without specific bond formation. Control experiments and different force profiles ( Supplementary Fig. 1 ) as well as electric double-layer interactions ( Supplementary Fig. 2 ) and statistics ( Supplementary Fig. 3 ) are discussed in detail in Supplementary Discussion 1 . Figure 2: Single-molecule force-induced rupture and force spectrum. ( a ) Typical non-equilibrium single-molecule rupture event measured in 1 mM NaCl, pH 6.5 at a pulling speed v p =0.25 μm s −1 . The approach and retract curves are indicated. The AFM zero distance, the distance to bond breaking D B as well as the contour length, L c (16.43 nm) of the used PEG tethers are indicated. Inset: About 100 pulling trajectories aligned with respect to pulling time using the best WLC-fit (red line, with persistence length as 3.65 Å). The scale bars are 2 nm and 5 ms. ( b ) Dynamic force spectra showing the logarithmic loading rate ( L R = v p k ) dependency of the unbinding force at pH=6.5. The near-equilibrium unbinding is visualized as a plateau for loading rates <10 5 pN s −1 . Non-equilibrium binding regimes are fit to the Bell–Evan’s equation as indicated by the solid line. The error bars represent s.e.m. Inset: histogram of breaking forces fitted to a Gaussian to extract the most probable unbinding force, F*. Full size image Figure 2b shows the loading rate dependency of the most probable rupture forces from which kinetic information about the transition state can be obtained from SM-AFM [8] , [17] . The force required for bond breaking increased upon increasing the loading rate as anticipated [17] . At lower loading rates, where the pulling rates fall close to the near-equilibrium regime, the breaking forces weakly depend on the pulling rate and plateau at 40–50 pN. At higher loading rates, Fig. 2b also indicates the kinetically different far-from-equilibrium regime where the irreversible rupture force increases linearly with the loading rate. This linear part can be fit well to the Bell–Evans theory as illustrated in Fig. 2b . For this weak acid–base bond, the fit gives the two model parameters, the kinetic off-rate k off =610±60 s −1 , and the distance from the bound to the transition state x B =0.5±0.5 Å. Using Arrhenius equation with a pre-exponential factor [18] of kT h −1 and the experimentally measured k off , the barrier height of the transition state is estimated as 23±0.2 kT. Extracting single-molecule interaction free energies To calculate the thermodynamic free energy difference between the bound and unbound state based on these non-equilibrium measurements, we further used the widely celebrated Jarzynski’s equality (JE) [15] , [16] : The central theme of this equality lies in the fact that it derives equilibrium free energy differences from the fluctuations of work, W n obtained from any process, irrespective of how far it is experimentally probed away from equilibrium. On the basis of the experimental determination of a sufficiently large set of work measurements, the exponentially averaged work for n →∞ number of work trajectories is expected to provide an accurate estimate for thermodynamic free energy difference, using equation (1). Ever since Jarzynski’s non-equilibrium work theorem in 1997, there has been a number of articles that discuss the application of this equality to single-molecule experiments using optical tweezers or AFM to unfold/refold the molecule [19] , [20] , [21] , [22] , [23] . These experiments necessitate defining the displacement of the thermally fluctuating cantilever from its equilibrium position. Hence this facilitates to exactly express JE [24] in terms of the extended non-equilibrium work theorem, allowing to reconstruct the free energy landscape from the force-extension curves corresponding to the (un)folding events [19] . Single-molecule adhesion experiments with a well-defined zero-force calibration can be well described using the original form of JE, that is, equation (1), utilizing the mechanical work measured within single-molecule pulling cycles. Consequently, for our analysis, we start with the original expression of the non-equilibrium work theorem derived by Jarzynski (equation (1)) and compare the result to the estimate of the free energy difference using the extended Hummer/Szabo method [19] , [21] , [24] , [25] . First, we define the starting point of the work where the cantilever experiences no force during retraction while in contact with the surface. Along the direction of the retraction of the tip, stretching of the PEG chains until bond rupture measures the work performed by the system. Hence, the work here relates to the mechanical loading of a polymer that is bound to the AFM tip through an acid–base bond. This corresponds to the initial bound state at the contact where Δ F =0 and D =0. The end state is defined at the distance D > D B just after bond rupture where Δ F =0, with the PEG tether and AFM cantilever in their respective equilibrium unbound situation. In cases of observed bond rupture, the mechanical work done by the system is characterized by the area under the retract segment of force versus distance curve. By integrating of the area under single-molecule pulling profiles, the work done until the bond rupture was measured. The exponent of this work, , was then averaged for all the n number of rupture events to obtain the JE free energy difference, as estimate for the free energy difference Δ G 0 . 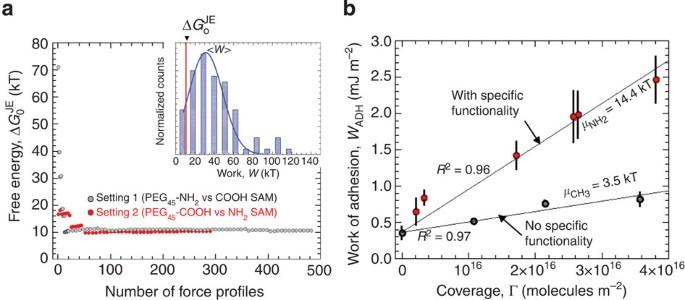Figure 3: Application of Jarzynski’s equality. (a) Evolution of the JE free energy for a series of unbinding events obtained with setting 1 and setting 2 respectively (cf.text for details). The inset shows the distribution of measured work. (b) Macroscopic work of adhesionWADHmeasured using SFA plotted against the tether coverage. The plotted data is for experiments with (PEG45–NH2) and without (PEG45–O–CH3) the possibility to form specific acid–amine bonds. Slopesμfitted from a linear model (W(Γ)=μ·Γ+WADH(Γ=0)) and correspondingR2values are indicated. Error bars represent s.d. The estimation can be expressed as Figure 3a shows the evolution of the JE free energy for a set of eight different experiments, and experimental settings and >1,000 different force profiles analysed using equation (2) at conditions close to and far from equilibrium. As can be seen from the figure, converges to 4.4e −20 ±0.1e −20 J, or 11±1 kT yielding a potentially very accurate estimate for the free energy difference Δ G 0 . As further shown in the inset in Fig. 3a , and as expected from the Clausius inequality (that is, < W >≥Δ G 0 ) the average of the work resulted in considerably higher interaction energies of 30–50 kT for these non-equilibrium experiments. Two aspects of our results are surprising: First, converges rapidly within the first 15–20 evaluated measurements, which we attribute to the fact that the measured bond is probed experimentally rather close to equilibrium in the first place. As can be seen in the classical Bell–Evans treatment (see Fig. 2b ), a wide plateau of the interaction force over the loading rate was measured for this particular system, indicating close-to-equilibrium conditions during bond rupture for most of the experimentally accessible loading rates. Here it is important to recognize that these are still non-equilibrium conditions, and hence a simple average of the work does not coincide with Δ G 0 . Also, experiments farther from equilibrium need a larger number of pulling cycles for full convergence. Second, the work distribution obtained in our measurements is rather broad and the estimate of the JE free energy may be largely biased by small values of the work, which are exponentially favoured by the JE treatment. Yet, the work distribution shown in Fig. 3a , indicates a good statistical sample with an expected energy within the lower end of the work distribution [16] . The obtained falls within the expected range of 5–15 kT for acid–base bonds in water [26] . Also, compares reasonably well to interaction free energies calculated for carboxylic acid–amine bonds in water using DFT-simulations [27] , and estimates for the interaction free energy of carboxylic acid cavitands with tertiary amines obtained by NMR [28] , which quote 6–17 kT and 5 kT, respectively. Figure 3: Application of Jarzynski’s equality. ( a ) Evolution of the JE free energy for a series of unbinding events obtained with setting 1 and setting 2 respectively ( cf. text for details). The inset shows the distribution of measured work. ( b ) Macroscopic work of adhesion W ADH measured using SFA plotted against the tether coverage. The plotted data is for experiments with (PEG 45 –NH 2 ) and without (PEG 45 –O–CH 3 ) the possibility to form specific acid–amine bonds. Slopes μ fitted from a linear model ( W (Γ)= μ ·Γ+ W ADH (Γ=0)) and corresponding R 2 values are indicated. Error bars represent s.d. Full size image To further test biasing of our estimates by small numbers, we also used the extended JE binning method [19] , [21] , [25] , which is not biased by small numbers. For this, force runs are aligned as a function of the total pulling time using the best worm-like chain fit. This allows to align the large number of measured single-molecule trajectories in terms of the initial time at Δ F =0 and D =0. The inset in Fig. 2a shows the resulting overlay of typical pulling curves (pulling velocity, v p =0.25 μm s −1 ) and the best WLC-fit, clearly indicating the breaking of an amine–acid bond bound through a PEG tether. The distance-dependent evolution of the Jarzynski sum, can be determined using the following equation [19] , [21] , [25] : where n is the total number of trajectories, z t is the displacement at any instance t , δ ( z − z t ) is the Dirac delta function and W n ( t ) is the mechanical work done in unbinding from time 0 to t . The values of obtained from this method are within 5% comparable to values obtained by applying equation (2) for the same corresponding set of force runs. Equation (3) involves reconstruction of the full bond-breaking free energy landscape, via aligning z coordinates in time before the exponential average is evaluated, which is physically and theoretically more meaningful. Equation (2) involves integrating the total area under the curve in terms of the mechanical work. Yet, the calculated free energy difference is very similar with both methods. It is interesting to mention that the AFM measurement shows a 10% error bar (that is, the progressive error over the set of >10 completely independent experiments for each setting), which we attribute mainly to the inaccuracy in determining the spring constant using the thermal noise method [29] . The variation due to the JE integration method used for extracting does not vary the error magnitude much. Yet, the binning method also allows for further extracting kinetic data from the JE treatment. This is yet to be fully explored [19] , [21] , [25] . Macroscopic adhesion force measurements using SFA To further experimentally assess the validity of the values obtained from the JE analysis of SM-AFM measurements, we compare the results from SM-AFM measurements with the equilibrium adhesion energy obtained from macroscopic measurements performed using the SFA. Based on its unique measuring principle [30] , the SFA has been used for almost three decades now to directly measure equilibrium free interaction energies [31] and may provide the ideal basis for evaluating the validity of the JE treatment of the SM-AFM data. With the SFA, macroscopic adhesion forces were measured as function of the number densities of PEG–NH 2 facing a COOH terminated SAM surface. Areal number densities of the PEG 45 –NH 2 in these experiments were varied over a bit more than one order of magnitude ranging from Γ=10 15 to 4 × 10 16 molecules per m 2 , where Γ refers to the coverage density. In this so-called mushroom regime [26] , the PEG chains are randomly distributed [32] , and do not interact significantly with each other. In Fig. 3b , the measured work of adhesion, obtained from the measured adhesion forces (see also Supplementary Fig. 4 and Supplementary Discussion 2 ) using Derjaguin–Müller–Toporov model [26] , F ADH =2 πRW ADH , is plotted against the number density of acid–amine bonds. The measured work of adhesion W tot (Γ) linearly scales with the number density Γ of potentially formed bonds, with the slope μ tot characterizing the total work of adhesion normalized per individual molecule, which amounts to 5.91e −20 J per molecule or 14.4±0.1 kT per molecule in the present case. It is important to note that our quantity of interest, that is, the slope does not depend on the actual contact model used. Here we use the Derjaguin–Müller–Toporov model because we do not observe contact deformation during detachment from the adhesive minimum, which is a direct observable in SFA measurements [30] . It is now interesting to separate effects due to the increase of the number density of acid–base bonds, and due to non-specific events such as backbone interactions, confinement of molecules between macroscopic SFA contact areas, or van der Waals and electric double-layer interactions. To perform control experiments that separate the backbone effects, selection of a non-specific terminal head group is crucial to avoid any undesirable interactions. Here, we have specifically chosen –O–CH 3 termination as it extends the alkyl chain (–O–CH 2 –CH 2 –O–) only by half a segment. Alternative terminations such as –OH termination would introduce the possibility to hydrogen bond specifically. Also, in comparison to the relatively long backbone chain, the density of the termination is lower and hence the non-specific contributions arising from the group itself can be considered negligible. Figure 3b also shows the non-specific work of adhesion W ns (Γ) measured during the separation of PEGolated surfaces with the methyl group termination. Hence, the slope μ ns of 1.45e −20 J per molecule or 3.5±0.1 kT per molecule indicates the background adhesion per individual backbone molecule. The difference μ specific = μ tot − μ ns of the slopes from experiments with and without functional group is hence the specific work of adhesion W specific (Γ) originating solely from acid–base bonds. This amounts to μ specific =10.9±0.2 kT per acid–base bond, and compares excellent with the interactions free energy obtained from AFM single-molecule force spectroscopy using JE. Hence, our measurements not only provide further experimental evidence proving the validity and practical applicability of JE, but also indicate that JE delivers the theoretical tool for unravelling macroscopic adhesion on the basis of non-equilibrium single-molecule adhesion measurements. In essence, these results suggest simple linear scaling relations for deciphering a large-scale adhesion event based on the molecular level details. In particular, the macroscopic work of adhesion W ADH per unit area may be calculated as a linear superposition of specific adhesion W specific , and non-specific, as well as scaling effects W ns as follows: The first term sums up the fraction x n of all specific single-molecular interactions (here only acid–base interactions with x n =1) in terms of the respective areal number densities Γ n . The second term W ns characterizes the additional work as linear superposition [26] of non-specific and background effects such as van der Waals (VDW) work of adhesion W VDW , the backbone interaction W MUSH or electric double-layer effects W EDL (see Supplementary Discussion 2 and Supplementary Table 1 ). It is important to emphasize, that some of the non-specific scaling effects such as the mushroom repulsion explicitly depend on the coverage, while others such as VDW forces are typically treated as integral and only implicitly depend on the coverage (for example, variation of the effective Hamaker constant due to different thin film dispersions [26] ). Also, some contribution may be attractive (VDW) and some may be repulsive ( W MUSH ). It is a matter of definition, whether or not one includes backbone interactions (that is, the mushroom repulsion) into the first part of the equation, which explicitly normalizes by the number density rather than by the total interacting area. The important conceptual aspect is the linear scaling relation, which does indeed hold. In fact, this term is not just a simple correction factor. On the basis of our approach, it is rather a measureable quantity. In the present case, the system was designed in such a way that the sum of the contributions from single-molecular specific adhesion events, plus all non-specific events indeed add up to the macroscopic value. As such, W ns (Γ) characterizes the work of adhesion without specific functionality in Fig. 3b characterizing all non-specific interactions. We tried to estimate the non-specific backbone binding energies using SM-AFM, however the measured forces are very close to and within the noise level of the AFM, and we cannot ascertain detection and correct integration of all events using SM-AFM potentially biasing evolution of the JE sum. In any case, it is beyond the scope of this work to decipher this part in detail as well. Table 1 summarizes all measured values. Table 1 Interaction free energy. Full size table Likewise, deconstructing any interacting system in such a way may be applicable to the most complex systems, with a number of different specific bonds interacting in parallel and may hence have important implications relevant to a wide range of fields and disciplines concerned with the macroscopic outcome of single-molecular events. All together, the presented approach also provides the perspective to study synergistic and antagonistic nonlinear scaling effects of multiple and different simultaneously interacting specific functionalities. By providing independent data for both sides of the equation, we present striking evidence that Jarzynski’s equality may be widely applicable even to quite broad work distributions given a large enough statistical sample. Hence JE provides the theoretical tool to understanding and predicting macroscopic equilibrium events based on the measurement of single-molecular non-equilibrium events. For the presented case of a simple bio-adhesive system with specific and non-specific interactions, we showed how the combination of SM-AFM and SFA measurements, as well as linear scaling relations based on JE, can detail macroscopic events and their scaling over up to seven orders of magnitude. Thus, force spectroscopy and SFA when used in direct conjunction with Jarzynski’s work theorem, will provide new insights into both exploring the energy landscapes of single bonds and the scaling behaviour of molecular interactions in a wide range of fields such as engineering and gluing, bio- and cell adhesion or molecular design of new functional materials. Likewise, the presented approach will allow testing the extrapolation of simulation studies to realistic scenarios found in living as well as engineering systems. Chemicals and materials All chemicals used were of the highest grade and were used without further purification (Supplier: Sigma Aldrich unless otherwise stated). The water was particle-free and filtered through a Milli-Q system. The lipids, 1,2-distearoyl-sn-glycero-3-phosphoethanolamine (DSPE), 1,2-distearoyl-sn-glycero-3-phosphoethanolamine-N-[carboxy(polyethylene glycol)-2000] ammonium salt (DSPE-PEG 45 -COOH), 1,2-distearoyl-sn-glycero-3-phosphoethanolamine-N-[amino(polyethylene glycol)-2000] ammonium salt (DSPE-PEG 45 –NH 2 ) and 1,2-distearoyl-sn-glycero-3-phosphoethanolamine-N-[methoxy(polyethylene glycol)-2000] ammonium salt (DSPE-PEG 45 –O–CH 3 ) were obtained from Avanti Lipids. Functionalization of AFM tips Rectangular gold-coated silicon cantilevers (CONTGB-G, BudgetSensors) were used. For the functionalization, we used the alkane thiols 11-Amino-1-undecanethiol hydrochloride and 11-Thiol-undecanoic acid. The gold-coated cantilevers were rinsed consecutively in 95 to 98% concentrated sulfuric acid (for 60 s), two batches of Milli-Q water, ethanol and were immediately submersed into freshly prepared 1 mM ethanolic solution of the alkane thiol. After a minimum of 12 h of exposure, the cantilevers were taken out of the solution, cleaned thoroughly with ethanol and a final rinse in hexane (~5 s) and ethanol, respectively to ensure the removal of unbound thiols, and dried in a stream of pre-purified nitrogen gas just before the force measurements. SAM formation was routinely checked with XPS. AFM tips were checked in SEM after every experiment (see Supplementary Fig. 1c ) to ensure stable tip geometry throughout the experiment. Details of our pre- and post-analysis, as well as functionalization standards can be found in the supporting information of Valtiner and Grundmeier [33] . Deposition of end-functionalized PEGolated lipid bilayers For bilayer deposition, both the lipids were suspended separately in a mixture of chloroform and methanol (7:3 volume fractions). The bilayer was deposited using Langmuir–Blodgett technique on a freshly cleaved mica surface glued to a glass-slide along with an o-ring using UV-curable glue (Norland Adhesive, NOA81). The inner layer of DSPE was transferred to the mica surface at the rate of 0.5 mm per min, at a lateral pressure of 40 mN m −1 and an area of 42 Å 2 per molecule [13] . For the outer layer, both DSPE and DSPE-PEG 45 –X (where X=COOH, NH 2 or –O–CH 3 ) were spread over the water sub-phase at a molar ratio of 0.1% and 0.5% of PEG 45 –X chains and deposited as described for the inner layer so that the spacing between adjacent PEG 45 –X molecules was 20 and 10 nm, respectively. The resultant bilayer as indicated in Fig. 1 was preserved under water without exposure to air using a fluid cell for the remainder of the experiment. This model system compares well with a cell membrane that extends specific tethers, in particular, PEG molecules are uniformly but randomly distributed over the surface area [13] , [34] , [35] . Supported PEGolated bilayers are well stable for the duration of a typically 6 h experiment, Kuhl et al . [13] quote a stability for more than 5 days. Also, we do not find degradation within the time scale of a typical experiment. The contour length of the chain of DSPE-PEG 45 was estimated as L c = n × L s =0.365 × 45=16.43 nm, where L s is the segment length of the PEG chain. Force spectroscopy All the experiments were performed in ambient electrolyte environments using a Nanowizard (JPK Instruments, Germany). The interactions were measured in a 1 mM NaCl solution whose pH was set to 6.5. The sensitivity of the AFM cantilever was measured through several force plots on the bilayer surface and compared with post-experimental measurements on a pristine mica surface to determine the error. The cantilever with self-assembled monolayer was calibrated to estimate its spring constant, k using thermal noise method. Typically the spring constants of different cantilevers varied from 250 to 500 pN nm −1 with sensitivity values from 65 to 100 nm V −1 . Applying the above information on the force runs, the cantilever deflection versus tip-sample separation distance was converted to force–distance profiles. D o =0, the apparent hard-wall was adjusted to the zero plane of the electrostatic double-layer interactions. Force runs were recorded at constant approach and pulling rate v P , while recording the force versus extension. The AFM was programmed to perform specific recognition mapping in a square grid pattern with 10 × 10 points separated at a distance of 20 or 10 nm, the same as the theoretical separation distance between the end-functionalized PEGolated lipid molecules for the given deposition conditions. The force runs were repeated 10 times on each point before moving to the subsequent one, thus collecting 1,000 individual force–distance curves per recognition map and loading rate to generate sufficient statistics. It was also programmed to approach the surface until a trigger force of F MAX =0.35 nN was reached to ensure the contact of the tip with the surface to pick single molecules. Higher approach forces were avoided to eliminate bilayer damage (see Supplementary Information ). For a given set of lipid concentration, the tip was retracted at various pulling speeds ranging from 50 nm s −1 to 1 μm s −1 on a logarithmic scale to acquire individual specific recognition maps of different loading rates. AFM data analysis All data were recorded and analysed using JPK data processing software. The different force profiles were categorized, sorted and probabilities of finding given characteristics were calculated. Worm-like chain fit or step-fit was applied to force profiles with characteristic bond rupture signatures [26] . In all the cases, the contour length was fixed to 16 nm and the breaking forces were read out. As customary, for dynamic force spectra ( Fig. 2b ), the s.e.m. is given as error. For all other values, the s.d. characterizes the given error bar. Interaction force measurements using the SFA SFA normal force measurements were performed at 21 °C in a clean room using the SFA 2000 model obtained from SurForce LLC (Santa Barbara, USA) [30] . Mica sheets used in these experiments were hand-cleaved to provide sheets with an area of several (typically 5–10) cm 2 and uniform thicknesses ranging from 2–5 μm. The edges of these sheets were melt-cut with a hot platinum wire. Particular care was taken to avoid contamination of the mica sheets by Pt-particles. By PVD, back-silvered mica sheets were cut into smaller pieces using a surgical blade, and were then glued to cylindrical silica disks with a nominal radius of curvature R =2 cm, using a UV-curable glue (Norland Adhesives, NOA81). Atomically smooth Au films and SAM-modified SFA discs were prepared by template stripping, as previously described [12] . Bilayers were deposited as described for AFM experiments. Bilayers were not allowed to dry or de-wet after deposition of the outer layer. Atomically smooth mica with respectively deposited PEGolated bilayers and molecularly smooth SAM-coated gold surfaces were mounted in the SFA in a cross cylinder configuration, creating a two-layer interferometer [36] . Absolute distance measurement and the surface geometry were measured using white light multiple beam interferometry. For details, the reader is referred to earlier work [30] . Time and relaxation effects of this system were studied in detail elsewhere [12] ; here, we made sure that contact time effects have no role. In particular, surfaces were approached quasi-static into close contact with a compressive force of >10 mN m −1 . Work of adhesion was then measured on separation after total contact times between 5 and 10 min, after which adhesive forces did not increase further with longer contact times. It is worth mentioning that the SFA is a unique technique that provides equilibrated adhesion energies and direct information about failure mechanism. In particular, on the basis of consecutive force runs, one can identify if lipid pluck-out occurs [37] . Here, we observed no lipid pluck-out and stable adhesion over a set of consecutive force runs at a particular position. On the basis of binding energy ratio of lipid pluck-out ( of ~30 kT) and the measured specific binding energy the gradient of the pluck-out force is expected to be much larger compared with the force gradient for breaking at the specific binding [37] . Hence, the weakest link is clearly the acid–base bond. The contact reference was measured in dry Argon between mica and gold. D=0 is referenced to the contact between SAM (1.9 nm thickness) and hydrated bilayer ( T BL =7.5 nm). How to cite this article: Raman, S. et al . Deciphering the scaling of single-molecule interactions using Jarzynski’s equality. Nat. Commun. 5:5539 doi: 10.1038/ncomms6539 (2014).